Spectroscopic detection and state preparation of a single praseodymium ion in a crystal The narrow optical transitions and long spin coherence times of rare earth ions in crystals make them desirable for a number of applications ranging from solid-state spectroscopy and laser physics to quantum information processing. However, investigations of these features have not been possible at the single-ion level. Here we show that the combination of cryogenic high-resolution laser spectroscopy with optical microscopy allows one to spectrally select individual praseodymium ions in yttrium orthosilicate. Furthermore, this spectral selectivity makes it possible to resolve neighbouring ions with a spatial precision of the order of 10 nm. In addition to elaborating on the essential experimental steps for achieving this long-sought goal, we demonstrate state preparation and read out of the three ground-state hyperfine levels, which are known to have lifetimes of the order of hundred seconds. One of the exciting scientific challenges of modern times is the realization of sophisticated networks for storage, processing, read out and transport of quantum information [1] . The success of this ambitious plan relies on the availability of suitable materials, much in the same way that the properties of silicon have been decisive for the rapid advance of microelectronics. A particularly appealing quantum system would be one that gives simultaneous access to narrow optical transitions and long spin coherence times [2] while lending itself to on-chip photonics integration [3] . As a result, atom-like solid-state emitters such as semiconductor quantum dots and colour centres have attracted a great deal of attention, but influences from their host matrices continue to limit the degree of attainable coherence in each case. An ideal alternative platform is based on the 4f-intrashell transitions of rare earth ions, which are well shielded from their surroundings [4] . In fact, recent ensemble experiments have demonstrated the potential of this system for quantum information processing [5] , [6] , [7] ; however, attempts to detect single ions via narrow optical transitions have not been fruitful. A special feature of rare earth ions is that their 4f-shell transitions are shielded from their environment by closed outer shells, allowing for long coherence times [8] . Level 3 H 4 acts as the electronic ground state with three doubly degenerate hyperfine sublevels at frequency spacings of 10.19 and 17.3 MHz (ref. 9 ). Hole burning measurements have shown the lifetimes of these levels to be as long as 100 s (refs 10 , 11 ), and spin coherence times up to one minute have been recently reported [7] , [12] , [13] . The well-defined narrow optical transitions, long hyperfine coherence times and access to Λ-level schemes make rare earth ions highly attractive for quantum optics [5] , [6] , [7] . On the other hand, the long excited-state lifetimes and the resulting weak emission have restricted previous studies to ensembles. Indeed, faint fluorescence, photobleaching and irreproducibility seem to have hampered progress in a few isolated attempts that have been reported over more than two decades [14] , [15] , [16] , [17] , [18] . About a year ago, Kolesov et al. [19] presented a solid proof of detecting single Pr 3+ ions at room temperature. These authors considered the direct detection of single ions via 4f–4f transitions to be unfeasible and circumvented the long optical coherence times by exciting the ion to the 5d-band in a multiphoton process. The room-temperature operation of this pioneering work, however, does not allow addressing the narrow optical transitions and hyperfine levels of the ground state. Another very recent publication reports on electrical detection of erbium ions in a silicon nanotransistor structure at cryogenic temperatures [20] , but optical read out and integration in photonics networks were not accessible. Here, we show that the combination of cryogenic high-resolution laser spectroscopy with optical microscopy allows one to spectrally select [21] individual praseodymium ions in yttrium orthosilicate (Y 2 SiO 5 , also called YSO). In addition, we demonstrate state preparation and read out of the three ground-state hyperfine levels, which are known to have lifetimes of the order of hundred seconds. Basic spectroscopic characterization of Pr 3+ in YSO In our laboratory we chose to excite Pr 3+ to the 3 P 0 state because its lifetime of 1.95 μs is shorter than 166 μs for the 1 D 2 state, which has been used in the great majority of the published research [5] , [7] , [11] , [12] , [13] , [22] . 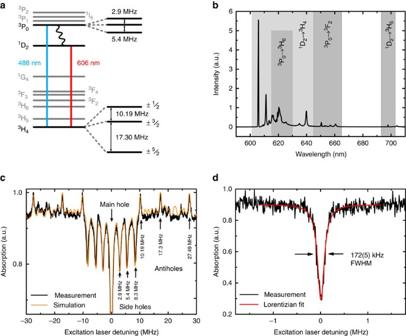Figure 1: Spectroscopic properties of Pr:YSO. (a) Level scheme of Pr3+in YSO. The ground (3H4) and excited states (3P0) show hyperfine splittings into three doubly degenerate levels. The hyperfine level splittings of3P0were measured for the first time in this report, but their spin assignments remain unknown. The spin values of the ground-state levels are displayed. (b) Fluorescence emission spectrum of bulk Pr:YSO with excitation light polarized parallel to the D1axis measured atT=4.3 K. The main peak at 606 nm corresponds to the transition from1D2to3H4. The spectral features at longer wavelengths correspond to transitions from either3P0or1D2to other intermediate levels as indicated. (c) Hole burning spectrum measured on an ensemble of Pr3+in a bulk YSO crystal. Side holes and anti-holes mark the excited and ground state hyperfine splittings, respectively. The orange spectrum presents a simulation (not a fit), assuming equal transition rates (see text). (d) Zoom of the main spectral hole at low-fluence excitation. Figure 1a sketches some of the energy levels of Pr 3+ in the visible spectrum while Fig. 1b provides more details on the emission spectrum. The correspondingly broader natural linewidth of 82 kHz instead of 1 kHz sets a less-stringent requirement for the bandwidth of the laser to be used. When an ion is excited to the 3 P 0 state, it can decay into each of the three ground state hyperfine levels via different pathways. The main channel involves a non-radiative relaxation to the 1 D 2 state followed by fluorescence decay at a wavelength of 606 nm. In our work, we used long-pass filters to collect the fluorescence at wavelengths above 595 nm. Figure 1: Spectroscopic properties of Pr:YSO. ( a ) Level scheme of Pr 3+ in YSO. The ground ( 3 H 4 ) and excited states ( 3 P 0 ) show hyperfine splittings into three doubly degenerate levels. The hyperfine level splittings of 3 P 0 were measured for the first time in this report, but their spin assignments remain unknown. The spin values of the ground-state levels are displayed. ( b ) Fluorescence emission spectrum of bulk Pr:YSO with excitation light polarized parallel to the D 1 axis measured at T =4.3 K. The main peak at 606 nm corresponds to the transition from 1 D 2 to 3 H 4 . The spectral features at longer wavelengths correspond to transitions from either 3 P 0 or 1 D 2 to other intermediate levels as indicated. ( c ) Hole burning spectrum measured on an ensemble of Pr 3+ in a bulk YSO crystal. Side holes and anti-holes mark the excited and ground state hyperfine splittings, respectively. The orange spectrum presents a simulation (not a fit), assuming equal transition rates (see text). ( d ) Zoom of the main spectral hole at low-fluence excitation. Full size image Considering the long lifetime of the ground state hyperfine levels, excitation at only one laser frequency would quickly transfer the population of any of the hyperfine levels into the other two. The resulting population trapping leads to the inhibition of fluorescence and is the mechanism that allows spectral hole burning [10] , [11] . In Fig. 1c we display an example of a hole-burning spectrum obtained from a bulk crystal at T =4.3 K. Here, a strong narrow-band laser beam at a fixed frequency was used to optically pump the population from one of the 3 H 4 hyperfine levels of a subclass of ions, thus ‘burning’ a spectral hole in the absorption profile of the sample. A weak probe laser was subsequently scanned over the spectral hole to report on the homogeneous broadening and the separation of the hyperfine levels. The spectral dips on the sides of the central hole in Fig. 1c reveal the hyperfine splittings of the 3 P 0 state at 2.9 MHz and 5.4 MHz, measured for the first time in Pr:YSO. The anti-holes appear at the expected frequency spacings of 10.19 MHz and 17.3 MHz for the hyperfine levels of the ground state [9] . The observed spectral features with linewidths of ~172 kHz in low-fluence hole-burning experiments ( Fig. 1d ) are consistent with a homogeneous width of 82 kHz and a laser linewidth below 10 kHz (see Methods section). Repeated scans verify that the hole depth and spectral position persist in the bulk sample for minutes, pointing to the absence of noticeable spectral diffusion in this system. The orange spectrum overlaid on the experimental hole-burning data presents a simulation, assuming equal weights for all nine possible transition rates involved in the 3 H 4 – 3 P 0 transition and neglecting other intermediate states. This simplified assumption yields very good agreement with the measurements, but a quantitative assignment of the transition rates requires detailed spectroscopic studies that go beyond the scope of this work. Detection of single ions via spectral selection To detect single ions on a low background, it is desirable to reduce the observation volume and ion concentration by as much as possible. In our current work, we were restricted to commercially available Pr:YSO crystals with minimum doping of 0.005%. Therefore, we milled a small piece of such a crystal to obtain micro- and nanocrystals. As sketched in Fig. 2a , the crystallites were deposited on the flat side of a cubic zirconia solid immersion lens (SIL) with a refractive index of n =2.15. The SIL was thermally contacted to a cold finger in a liquid helium flow cryostat. A continuous-wave Ti:sapphire laser operating at 976 nm was locked to a high-finesse cavity to achieve a spectral linewidth below 10 kHz and long-term spectral stability ( Fig. 2b ). For addressing the 3 H 4 – 3 P 0 transition, the resulting laser light was frequency doubled to 488 nm in a resonant cavity and could be scanned over 600 MHz using an acousto-optical modulator (AOM) in double-pass mode. Broader spectral investigations could be obtained by stitching these scans. The laser beam was then coupled to a microscope objective (numerical aperture 0.75) that was scanned by a three-dimensional (3D) piezoelectric actuator. We used a single-photon detector with very low dark counts to measure the fluorescence signal from the sample in reflection and employed another avalanche photodiode (APD) to detect the laser light in transmission through a bore in the cold finger. 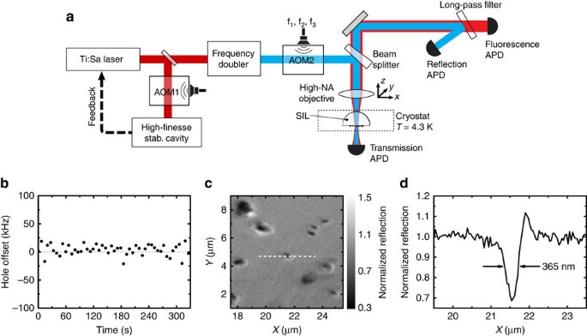Figure 2: Experimental setup and reflection scan image. (a) Schematic of the experimental setup. A frequency-stabilized Ti:sapphire laser is frequency-doubled and used for excitation. An acousto-optical modulator (AOM1) scans the frequency of the fundamental light. A second modulator (AOM2) produces the three frequenciesf1,f2andf3described in the main text. Pr:YSO microcrystals are placed on the flat side of a hemispherical SIL inside a liquid helium flow cryostat. The 488-nm excitation light is focused onto the microcrystals by a high-NA objective mounted on a 3D piezo stage. Fluorescence and the reflected light are detected through the same objective. (b) Position of the spectral hole centre after a single burn pulse and repeated scans. The measurement confirms the long-term frequency stability. (c) Reflection scan image of the sample, visualizing the individual micro- and nanocrystals. (d) Cross section of the nanocrystal used in our measurements taken from the scan image in (c). Figure 2: Experimental setup and reflection scan image. ( a ) Schematic of the experimental setup. A frequency-stabilized Ti:sapphire laser is frequency-doubled and used for excitation. An acousto-optical modulator (AOM1) scans the frequency of the fundamental light. A second modulator (AOM2) produces the three frequencies f 1 , f 2 and f 3 described in the main text. Pr:YSO microcrystals are placed on the flat side of a hemispherical SIL inside a liquid helium flow cryostat. The 488-nm excitation light is focused onto the microcrystals by a high-NA objective mounted on a 3D piezo stage. Fluorescence and the reflected light are detected through the same objective. ( b ) Position of the spectral hole centre after a single burn pulse and repeated scans. The measurement confirms the long-term frequency stability. ( c ) Reflection scan image of the sample, visualizing the individual micro- and nanocrystals. ( d ) Cross section of the nanocrystal used in our measurements taken from the scan image in ( c ). Full size image The first step of our measurements consisted of imaging individual YSO crystallites on the SIL surface. Here, we monitored the reflected excitation light on a photodetector to record the interference between the light fields scattered by the small crystals and the SIL surface. Figure 2c displays a scanning image of the crystallites using this interferometric scattering (iSCAT) contrast, which depends on the size and index of refraction of the object under illumination [23] . For the experiments discussed below, we used the nanocrystal in the middle of the image, which we estimate from the cross-section in Fig. 2d to be of the order of 100–200 nm in size. Considering the weak signal of an ion, even small sample drifts can complicate the measurements. We, thus, used the iSCAT signal to also actively lock the laser spot to the nanocrystal, making it possible to study a single ion for hours. To avoid population trapping in the hyperfine levels of the ground state, we used a second AOM to generate two frequencies at f 1 = f 2 −10.19 MHz and f 3 = f 2 +17.3 MHz in addition to the laser frequency ( f 2 ). This allowed us to simultaneously excite all three hyperfine levels of the ground state. 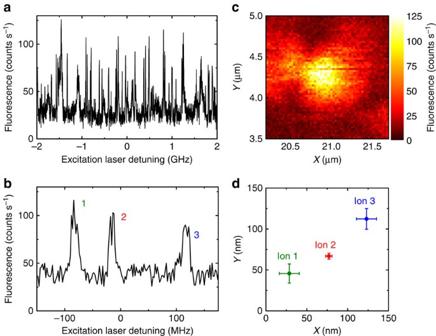Figure 3: Spectral detection and spatial localization of single ions. (a) Fluorescence excitation spectrum recorded at the speed of 1 MHz s−1over several GHz. Narrow resonances are attributed to single ions. (b) An excitation fluorescence spectrum recorded over ~300 MHz, consisting of three ions. (c) Laser scanning fluorescence image of a single ion recorded on resonance. (d) Super-resolution colocalization image of the three ions detected in (b). The error bars depict the standard error of the mean ion position, calculated from eight measurements per ion. Figure 3a shows an example of an excitation fluorescence spectrum when frequencies f 1 , f 2 and f 3 were scanned over 4 GHz. To reduce the measurement time, this spectrum was recorded with a laser linewidth of ~1 MHz without using external cavity locking. A background fluorescence as low as ~20–30 counts per second allows the detection of narrow spectral features. Figure 3b plots a zoom into three narrow resonances recorded with the narrow-band laser (<10 kHz). In most cases, such peaks were spectrally stable over measurement times of the order of hours although we also observed some spectral jumps. The sparse appearance of the observed narrow spectral lines lets us attribute them to the emission of single Pr 3+ ions [21] . Figure 3: Spectral detection and spatial localization of single ions. ( a ) Fluorescence excitation spectrum recorded at the speed of 1 MHz s −1 over several GHz. Narrow resonances are attributed to single ions. ( b ) An excitation fluorescence spectrum recorded over ~300 MHz, consisting of three ions. ( c ) Laser scanning fluorescence image of a single ion recorded on resonance. ( d ) Super-resolution colocalization image of the three ions detected in ( b ). The error bars depict the standard error of the mean ion position, calculated from eight measurements per ion. Full size image Super-resolution imaging of ions Each of the spectrally detected ions can be spatially mapped in fluorescence. Figure 3c presents a laser-scanning image of the fluorescence signal when the laser frequency was tuned to a narrow resonance. Fitting the image of the diffraction-limited spot lets us localize the ion with a precision of the order of 10 nm. By repeating this procedure for each resonance, one can colocalize all the ions in the sample beyond the diffraction limit. Figure 3d illustrates this idea for the three ions of Fig. 3b . Combination of this type of super-resolution microscopy and high-resolution spectral data will open the way for quantitative studies of near-field coupling among several ions [24] . The effect of excited-state hyperfine levels Up to this point, we treated the excited state as one level. However, one has to bear in mind that the 3 P 0 state consists of three hyperfine levels at separations of 2.9 and 5.4 MHz ( Fig. 1c ), which become resonant with the three laser frequencies f 1 , f 2 and f 3 at different detunings. The blue spectrum in Fig. 4a plots the fluorescence signal that is expected from coupling the three ground-state hyperfine levels to the three excited-state hyperfine levels if one assumes a linewidth of 82 kHz. The three peaks occur whenever the laser detuning matches the transition of all ground state hyperfine levels to one of the excited state hyperfine levels. They are not affected by population trapping in one of the ground states. The displayed spectrum was calculated using a simple rate equation model, where the ion was described as a six-level system (see Methods section). 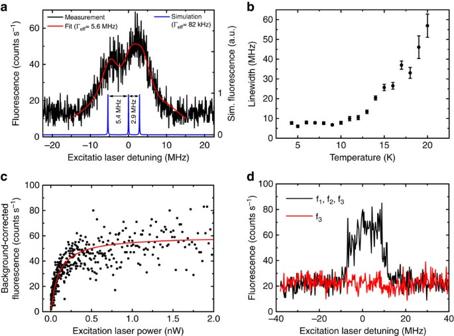Figure 4: Some spectroscopic features of a single ion. (a) The blue trace depicts a simulated spectrum, assuming a transition linewidth of 82 kHz. The black curve plots an experimental high-resolution excitation spectrum of a single ion sampled at 0.1 s and averaged over 10 traces. The substructure originating from the excited state hyperfine splitting is clearly visible. The red curve displays a fit, assuming a full width at a half-maximum of 5.6 MHz. (b) Temperature dependence of the full width at half-maximum of the resonance, neglecting the underlying structure of the three hyperfine transitions. The error bars indicate the fit uncertainty of the Lorentzian linewidth. (c) Background-corrected fluorescence of a single ion as a function of the excitation power. The red curve denotes a fit assuming a three-level system. (d) Fluorescence signal recorded when addressing all hyperfine levels of the ground state (black) compared with the case where only the lower level was excited (red). In the latter case, population is trapped in the higher hyperfine levels. Figure 4: Some spectroscopic features of a single ion. ( a ) The blue trace depicts a simulated spectrum, assuming a transition linewidth of 82 kHz. The black curve plots an experimental high-resolution excitation spectrum of a single ion sampled at 0.1 s and averaged over 10 traces. The substructure originating from the excited state hyperfine splitting is clearly visible. The red curve displays a fit, assuming a full width at a half-maximum of 5.6 MHz. ( b ) Temperature dependence of the full width at half-maximum of the resonance, neglecting the underlying structure of the three hyperfine transitions. The error bars indicate the fit uncertainty of the Lorentzian linewidth. ( c ) Background-corrected fluorescence of a single ion as a function of the excitation power. The red curve denotes a fit assuming a three-level system. ( d ) Fluorescence signal recorded when addressing all hyperfine levels of the ground state (black) compared with the case where only the lower level was excited (red). In the latter case, population is trapped in the higher hyperfine levels. Full size image The spectra in Fig. 3b do not mirror the expected multitude of narrow resonances in Fig. 4a , but spectra recorded at higher sampling resolution (see black curve in Fig. 4a ) clearly show a substructure. We attribute this broadening to spectral diffusion caused by the strain in the milled crystallites. The red curve shows that the measured spectrum in Fig. 4a can be matched if we consider the individual transitions to be broadened to 5.6 MHz. We point out that although size-related deviations of the linewidth are expected in very small nanocrystals [25] , there is no fundamental reason for the existence of dephasing in crystallites. Proper preparation and handling can minimize [26] or eliminate spectral diffusion. Furthermore, as shown in Fig. 4b , we have verified that the observed linewidths are not limited by temperature. Figure 4c plots the fluorescence signal at the peak of a recorded resonance as a function of the excitation power. We report a measured saturation power of 98 pW in each of the three laser beams equivalent to an intensity of I sat ≈46 mW cm −2 . We point out, however, that this is an approximate value because the overlapping broad transitions of various hyperfine levels make it difficult to assign a well-defined saturation power. The measurement also indicates a maximum detected count rate of ~60 photons per second. This is 6–8 times smaller than the count rate of 350–500 photons per second predicted by rate equations, when taking into account the upper 3 P 0 , intermediate 1 D 2 and ground state 3 H 4 , as well as our measured detection efficiency of 11% and estimated collection efficiency of ~54–78% through the SIL (see Methods section). One possible explanation for this discrepancy is the existence of a transition to a long-lived state at energies below the 1 D 2 state ( Fig. 1a ), which could act as bottle neck. Although the branching ratio of decay into such a state can be moderate ( Fig. 1b ), a lifetime of the order of 500 μs, which is typical for 4f-shell transitions, would suffice to rectify the observed discrepancy (see also discussion in Methods section). It should be noted that proper optical pumping out of these trap states would allow one to recover the maximum fluorescence rate. Earlier we argued that we needed three laser frequencies to prevent shelving in various hyperfine levels of the ground state. While Fig. 4d verifies this statement, the black spectra in Fig. 5a–c illustrate that the fluorescence survives if one turns off one of the frequency components f 1 , f 2 or f 3 . To understand this observation, we simulated the excitation and fluorescence dynamics of the ion, using equally weighted branching ratios (as in the simulation shown in Fig. 1c ). The blue traces in Fig. 5a–c show that one would expect very faint peaks for transition linewidths of 82 kHz. However, larger homogeneous linewidths make the various transitions overlap so that all three ground states can be partially addressed with only two laser frequencies. As a result, strict population trapping is avoided. Indeed, the fits in Fig. 5a–c presented by the red solid curves indicate that the recorded experimental data can be reproduced if a homogeneous linewidth of 3.3 MHz is assumed for this ion (different from the one examined in Fig. 4a ). The simulated spectra in Fig. 5a–c also reveal that the influence of the transition linewidth on population trapping leads to a nontrivial effect on the line shapes. In Fig. 5a , for example, the most prominent spectral peak for the linewidth of 3.3 MHz is due to f 3 depopulating the lowest ground state, while f 2 depopulates the two higher lying ground states. 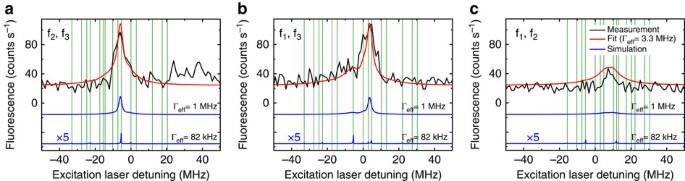Figure 5: Two-frequency response. (a–c), Excitation spectra of a single ion illuminated by different combinations of only two laser frequencies. The legend in each plot denotes the frequencies that were turned on. The vertical green lines indicate the potential transitions for the given two-frequency excitation. The red curves were obtained by fitting all three experimental two-frequency spectra (black) simultaneously. The blue curves are simulations assuming interaction linewidths of 1 MHz and 82 kHz and are downshifted for better visibility. The zero of the horizontal axis denotes the frequency at whichf2becomes resonant with the centre hyperfine levels of the ground and excited states. Figure 5: Two-frequency response. ( a – c ), Excitation spectra of a single ion illuminated by different combinations of only two laser frequencies. The legend in each plot denotes the frequencies that were turned on. The vertical green lines indicate the potential transitions for the given two-frequency excitation. The red curves were obtained by fitting all three experimental two-frequency spectra (black) simultaneously. The blue curves are simulations assuming interaction linewidths of 1 MHz and 82 kHz and are downshifted for better visibility. The zero of the horizontal axis denotes the frequency at which f 2 becomes resonant with the centre hyperfine levels of the ground and excited states. Full size image State preparation and read out The above measurements illustrate that a single ion can be prepared in a selected ground state by continuous optical pumping of the population to the desired state. To demonstrate the read out of the resulting quantum states, we implemented a pulsed excitation scheme sketched in Fig. 6a . The pulses were generated by a digital delay and a pulse generator and were applied independently to the three laser lines by the same AOM that produced f 1 , f 2 and f 3 . Two laser frequencies were turned on to pump the population out of two hyperfine levels to the third one. The pump duration of 344 μs was chosen to reach a population transfer of ~90%. A delay of 378 μs was implemented to allow the ion to decay from the excited state before applying the read-out pulse of 378 μs at the frequency of the third hyperfine level. This pulse drove the population for a few cycles until it was again trapped in the other two levels. We applied a gate pulse during the read out to discriminate against background and preparation pulse counts. 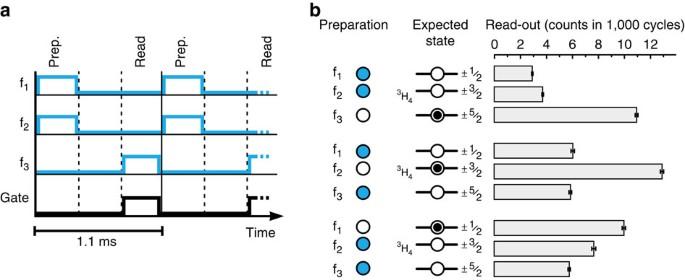Figure 6: State preparation and read-out. (a) An example of a pulse sequence for state preparation and read-out of a single ion. The ion is pumped into one of the hyperfine levels by two laser frequencies that are resonant with the other two hyperfine levels. A single laser frequency is used for the read out. (b) Three different scenarios for preparing the ion in the lowest, middle or upper hyperfine levels of the ground state (spin values are displayed in each case). In all three cases, the read-out clearly shows a high-fluorescence yield only when the read-out laser is resonant with the previously populated hyperfine level. Each sequence was cycled for 100 s to obtain a sufficient signal-to-noise ratio. The error bars show the standard error of the mean counts in 1,000 cycles, at the respective preparation and read-out configuration. Figure 6b displays the outcome of three sets of such measurements over 100 s. It is clear that if the read-out pulse is resonant with the state in which the ion was prepared, the fluorescence signal is maximized. These data exhibit the ease with which a single rare earth ion can be optically prepared in a hyperfine level of the electronic ground state, although in the current investigation the preparation efficiency was compromised due to the broadening and overlaps of the transitions. Figure 6: State preparation and read-out. ( a ) An example of a pulse sequence for state preparation and read-out of a single ion. The ion is pumped into one of the hyperfine levels by two laser frequencies that are resonant with the other two hyperfine levels. A single laser frequency is used for the read out. ( b ) Three different scenarios for preparing the ion in the lowest, middle or upper hyperfine levels of the ground state (spin values are displayed in each case). In all three cases, the read-out clearly shows a high-fluorescence yield only when the read-out laser is resonant with the previously populated hyperfine level. Each sequence was cycled for 100 s to obtain a sufficient signal-to-noise ratio. The error bars show the standard error of the mean counts in 1,000 cycles, at the respective preparation and read-out configuration. Full size image High-resolution spectroscopy of rare earths at the single-ion level combined with microscopy and magnetic resonance spectroscopy [7] , [22] , [27] would provide unprecedented opportunities for exploring fundamental phenomena such as dipole coupling, energy transfer and phonon broadening in materials of technological relevance [4] without the ambiguities associated with ensemble inhomogeneities. Furthermore, our results stimulate new experimental frontiers for quantum information science [1] , [2] . In particular, on-chip nanoscopic waveguides and interferometers [3] made of Pr:YSO could offer an ideal platform for connecting atom-like qubits via efficient photonic channels. The only shortcoming of the rare earth systems, namely their weak emission that led many groups to consider their direct detection to be unfeasible via the 4f-shell transitions [19] , can be readily improved in future works. First, higher collection [28] and detection efficiencies could increase the fluorescence count rates to several thousand counts per second. Moreover, the spontaneous emission rate and branching ratios can be modified by hundreds to thousands times via application of microcavities [29] and nano-antennas [30] . We hope that our work inspires further activities towards the detection of single ions also in other guest–host systems. Spectral hole burning For the spectral hole-burning experiments we replaced the microscope objective by a lens with focal length f =300 mm in order to interact with a multitude of ions under a uniform illumination. The excitation light was re-collimated behind the cryostat and sent to the detector. We tuned the laser to the centre of the inhomogeneous broadening and burnt a spectral hole with a short but intense laser pulse using only a single laser frequency. To interrogate the spectral hole, the laser intensity was strongly reduced and the frequency was scanned over the hole while recording the transmitted signal. Before commencing the next cycle, the hole was cleared by heating the sample to 12 K and subsequently cooling to 4.3 K. The hole-burning spectrum in Fig. 1c of the main article is an average of 15 scans. The burn pulse had ~5 μW for 100 ms, and the scan was performed with 25 nW over a scan range of 60 MHz within 20 s. The strong burn fluence led to the power broadening of the centre hole. To get around this, we repeated the experiments with a burn pulse of only 160 nW for 200 ms and subsequently scanned the laser with 0.7 nW in 500 ms over 4 MHz. Figure 1d in the main text shows an average of 20 scans of the centre hole measured at low fluence. A Lorentzian fit to the hole yields a FWHM of 172 kHz. Since a laser beam with linewidth Γ laser interacts with transitions of linewidth Γ hom during the burn and scan sequence, the total hole width is given by Γ hole =2(Γ laser +Γ hom ). Accounting for the homogeneous linewidth of Γ hom =82 kHz deduced from lifetime measurements, we estimate a laser linewidth of 4±2.5 kHz. In order to estimate the long-term laser frequency stability, we burnt a hole with a high fluence to achieve a good signal-to-noise ratio and repeatedly scanned the hole for several minutes (without heat and re-cool cycles). Each scan was fitted with a Lorentzian to determine the hole centre frequency as a function of time. Long-term drifts of the laser frequency would lead to a shift of the hole position while dephasing in the sample would result in a broadening and reduction of the hole depth. Figure 2b displays the hole centre distribution over 6 min in 7-s intervals. The fit uncertainty of the hole centres is 6 kHz. Together with the standard deviation of the data points (9 kHz) we can estimate the frequency stability to be on a time scale of 7 s. A further drift on the scale of minutes is not observable. This is also confirmed by the spectral stability of the single ion resonances in consecutive scans. Simulation of the excitation spectra For a better understanding of the single ion fluorescence, we set up a rate equation model, where the ion is described as a six-level system, taking into account the three ground and three excited hyperfine states, neglecting the intermediate state 1 D 2 . The values of the hyperfine splittings are taken from hole-burning measurements and no population transfer within the manifolds of the excited or ground states is allowed. The transfer from the ground to the excited state is driven by the laser frequencies with the splittings of 10.19 MHz and 17.3 MHz, which are scanned synchronously. In this simple model, each transition is taken to be Lorentzian. Maximum emission rate at saturation To model the saturation behaviour of an ion, we first assume a rate-equation model involving the ground state 3 H 4 , the excited state 3 P 0 and the intermediate state 1 D 2 . The decay from 3 P 0 to 1 D 2 and 3 H 4 is modelled according to the branching ratios, which were determined from fluorescence spectra (such as Fig. 1b ) to be 3 P 0 → 1 D 2 =39%. The decay rates of 3 P 0 and 1 D 2 were chosen according to the experimentally measured values of 1.95 μs and 166 μs, respectively. This simple model predicts a photon rate of ~5,800 photons per second emerging from the 1 D 2 → 3 H 4 transition at saturation. To estimate the detectable count rate, both the collection efficiency of the objective and the detection efficiency of the setup have to be taken into account. The former can be estimated from calculations [31] . The refractive index contrast alters the dipole emission pattern such that a larger fraction of the photons is emitted into the solid angle visible to the objective. We assume an interface between the SIL and air, with a refractive index contrast of n SIL / n air =2.15, and place the emitter in the low-index medium. To account for the crystal size, the distance to the high-index medium is set to 50 nm. For a collection numerical aperture of 0.75, this results in a collection efficiency of 78% for dipole moments parallel to the SIL interface, and 54% for orthogonal dipole moments. Since the orientation of the dipole with respect to the interface is not known in a nanocrystal sample, we take the collection efficiency to be between 54 and 78%. The detection efficiency was measured to be 11% by examining the transmission of a laser beam from the objective to the detector at the emission wavelength. This figure also includes the 25% quantum efficiency of the APD. In total, we deduce the maximum detected count rate to be 5,800 × 0.11 × (0.54 to 0.78)=350 to 500 photons per second. We believe the reason for the observed lower emission rate of 60 counts per second is decay into the intermediate states such as 3 H 6 , 3 H 5 , 3 F 2,3,4 , 1 G 4 lying in between 1 D 2 and 3 H 4 . Long lifetimes of these states can lead to population trapping and lower emission at saturation [19] . Since little is known about the intermediate states in the literature, we introduce a fourth state in the rate equations to represent their combined effect. Using a more differentiated account of the recorded emission spectra in a bulk crystal, we determined the branching ratios to be 3 P 0 → 1 D 2 =39%, 3 P 0 → 3 H 4 =13% and 3 P 0 → 3 H 6 / 3 H 5 / 3 F 2,3,4 =48%. All decays from the intermediate states were assumed to be invisible to the detection. The lower measured count rates can be explained if one assumes a lifetime of the order of 500 μs for this effective fourth state. Although concrete experimental data are rare on our system, this estimate is a realistic order of magnitude for rare earth ions. In particular, calculations suggest that 1 G 4 might be involved [32] . How to cite this article: Utikal, T. et al. Spectroscopic detection and state preparation of a single praseodymium ion in a crystal. Nat. Commun. 5:3627 doi: 10.1038/ncomms4627 (2014).